Robust classification of salient links in complex networks Complex networks in natural, social and technological systems generically exhibit an abundance of rich information. Extracting meaningful structural features from data is one of the most challenging tasks in network theory. Many methods and concepts have been proposed to address this problem such as centrality statistics, motifs, community clusters and backbones, but such schemes typically rely on external and arbitrary parameters. It is unknown whether generic networks permit the classification of elements without external intervention. Here we show that link salience is a robust approach to classifying network elements based on a consensus estimate of all nodes. A wide range of empirical networks exhibit a natural, network-implicit classification of links into qualitatively distinct groups, and the salient skeletons have generic statistical properties. Salience also predicts essential features of contagion phenomena on networks, and points towards a better understanding of universal features in empirical networks that are masked by their complexity. Many systems in physics, biology, social science, economics and technology are best modelled as a collection of discrete elements that interact through an intricate, complex set of connections. Complex network theory, a marriage of ideas and methods from statistical physics and graph theory, has become one of the most successful frameworks for studying these systems [1] , [2] , [3] , [4] , [5] , [6] , [7] and has led to major advances in our understanding of transportation [8] , [9] , [10] , [11] , ecological systems [12] , [13] , social and communication networks [14] and metabolic and gene regulatory pathways in living cells [15] , [16] , [17] . One of the challenges in complex network research is the identification of essential structural features that are typically masked by a network's complexity [1] , [6] , [18] , [19] , [20] . Reducing a large-scale network to its core components, filtering redundant information and extracting essential components are not only critical for efficient network data management. More importantly, these methods are often required to better understand evolutionary and dynamical processes on networks and to identify universal principles of network design or growth. In this context, the notion of centrality measures according to which nodes or links can be ranked is fundamental and epitomized by the node degree k , the number of directly connected neighbours of a node. Many systems, ranging from human sexual contacts [21] to computer networks [22] , are characterized by a power-law degree distribution p ( k ) ∼ k −(1+ β ) with an exponent 0< β ≤2. These networks are scale-free [23] , meaning the majority of nodes are weakly connected and dominated by a few strongly connected nodes, known as hubs. Although a variety of networks can be understood in terms of their topological connectivity (the set of nodes and links), a number of systems are better captured by weighted networks in which links carry weights w that quantify their strengths [8] , [24] . An important class of networks exhibit both a scale-free degree distribution and broadly distributed weights, which in some cases follow a power-law p ( w ) ∼ w −(1+ β ) , with 1< α ≤2. [25] , [26] , [27] In addition to hubs, these networks thus possess highways. Several representative networks of this class are depicted in Fig. 1 . Understanding the essential underlying structures in these networks is particularly challenging because of the mix of link and node heterogeneity. 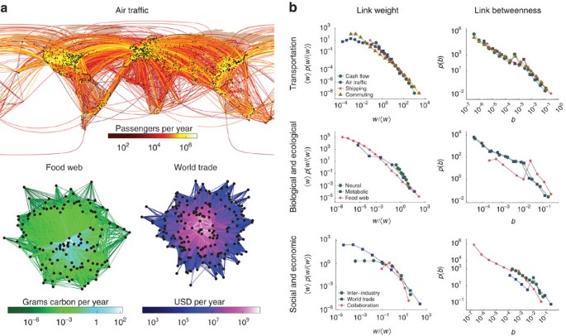Figure 1: Generic statistical properties of heterogeneous complex networks. (a) Geographical representation of the worldwide air traffic network (top), black dots represent airports, links represent passenger flux between them, link weightswijare colour encoded from dark (weak) to white (strong). Networks on the lower left and right represent the Florida Bay food web and the World trade network, respectively. Nodes in the food web are species and links represent the exchange of biomass; in the trade network nodes are countries and links quantify exchange in assets measured in USD. (b) Relative frequenciesf(w)=kwlp(w/kwl) andp(b) of link weightswand link betweennessbof representative transportation, biological, ecological, social, and economic networks. Link weights are normalized by the mean weight kwl. Details on each network are provided in Methods. In all networks link weights and betweenness are distributed across many orders of magnitude, and both statistics exhibit heavy tails. The substantial variability in these quantities is also reflected in their coefficient of variation (seeTable 1). Figure 1: Generic statistical properties of heterogeneous complex networks. ( a ) Geographical representation of the worldwide air traffic network (top), black dots represent airports, links represent passenger flux between them, link weights w ij are colour encoded from dark (weak) to white (strong). Networks on the lower left and right represent the Florida Bay food web and the World trade network, respectively. Nodes in the food web are species and links represent the exchange of biomass; in the trade network nodes are countries and links quantify exchange in assets measured in USD. ( b ) Relative frequencies f (w)=k wlp ( w /k w l) and p ( b ) of link weights w and link betweenness b of representative transportation, biological, ecological, social, and economic networks. Link weights are normalized by the mean weight k w l. Details on each network are provided in Methods. In all networks link weights and betweenness are distributed across many orders of magnitude, and both statistics exhibit heavy tails. The substantial variability in these quantities is also reflected in their coefficient of variation (see Table 1 ). Full size image Although classifications of network elements according to degree, weight or other centrality measures have been employed in many contexts [9] , [28] , [29] , [30] , this approach comes with several drawbacks. The qualitative concepts of hubs and highways suggest a clear-cut, network-intrinsic categorization of elements. However, these centrality measures are typically distributed continuously and generally do not provide a straightforward separation of elements into qualitatively distinct groups. At what precise degree does a node become a hub? At what strength does a link become a highway? Despite significant advances, current state-of-the-art methods rely on system-specific thresholds, comparisons to null models or imposed topological constraints [6] , [11] , [31] , [32] , [33] . Whether generic heterogeneous networks provide a way to intrinsically segregate elements into qualitatively distinct groups remains an open question. In addition to this fundamental question, centrality thresholding is particularly problematic in heterogeneous networks as key properties of reduced networks can sensitively depend on the chosen threshold. Here we address these problems by introducing the concept of link salience. The approach is based on an ensemble of node-specific perspectives of the network, and quantifies the extent to which a consensus among nodes exists regarding the importance of a link. We show that salience is fundamentally different from link betweenness centrality and that it successfully classifies links into distinct groups without external parameters or thresholds. On the basis of this classification, we introduce the high-salience skeleton (HSS) of a network and compute this structure for a variety of networks from transportation, biology, sociology and economics. We show that despite major differences between representative networks, the skeletons of all networks exhibit similar statistical and topological properties and significantly differ from alternative backbone structures such as minimal spanning trees. Analysing traditional random network models, we demonstrate that neither broad weight nor degree distributions alone are sufficient to produce the patterns observed in real networks. Furthermore, we provide evidence that the emergence of distinct link classes is the result of the interplay of broadly distributed node degrees and link weights. We demonstrate how a static and deterministic analysis of a network based on link salience can successfully predict the behaviour of dynamical processes. We conclude that the large class of networks that exhibit broad weight and degree distributions may evolve according to fundamentally similar rules that give rise to similar core structures. Link salience Weighted networks like those depicted in Fig. 1 can be represented by a symmetric, weighted N × N matrix W , where N is the number of nodes. Elements w ij ≥0 quantify the coupling strength between nodes i and j . Depending on the context, w ij might reflect the passenger flux between locations in transportation networks, the synaptic strength between neurons in a neural network, the value of assets exchanged between firms in a trade network or the contact rate between individuals in a social network. Our analysis is based on the concept of effective proximity d ij defined by the reciprocal coupling strength d ij =1/ w ij . Effective proximity captures the intuitive notion that strongly (weakly) coupled nodes are close to (distant from) each other [34] . It also provides one way to define the length of a path p that connects two terminal nodes ( n 1 , n k ) and consists of K −1 legs by a sequence of intermediate nodes n i , and connections The shortest path minimizes the total effective distance and can be interpreted as the most efficient route between its terminal nodes [35] , [36] ; this definition of shortest path is used throughout this paper. In networks with homogeneous weights, shortest paths are typically degenerate and many different shortest paths coexist for a given pair of terminal nodes. In heterogeneous networks with real-valued weights shortest paths are typically unique. For a fixed reference node r , the collection of shortest paths to all other nodes defines the shortest-path tree (SPT; T ( r )), which summarizes the most effective routes from the reference node r to the rest of the network. T ( r ) is conveniently represented by a symmetric N × N matrix with elements t ij ( r )=1 if the link ( i , j ) is part of at least one of the shortest paths and t ij ( r )=0 if it is not. The central idea of our approach is based on the notion of the average SPT as illustrated in Fig. 2a . 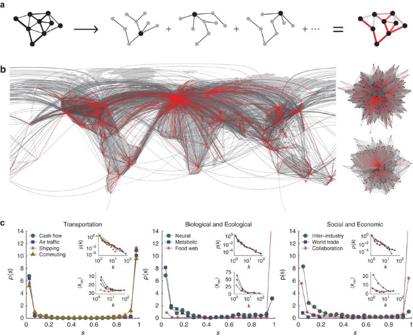Figure 2: Computation of link salience and properties of the HSS. (a) For each reference noderin the weighted network on the left, the SPTT(r) is computed. The superposition of all trees according to equation (1) assigns a valuesijto each link in the original network. Salience values are shown on the right with link colour: red is high salience and grey is low. (b) The collection of high-salience links (red) for the networks shown inFig. 1. The full networks are shown in grey. (c) The relative frequencyp(s) of non-zero salience valuess. The distributionp(s) is bimodal in all networks under consideration. This key feature of bimodality ofp(s) provides a plausible, parameter-insensitive classification of links, salient (s≈1) versus non-salient (s≈0), and implies that nodes in these networks typically agree whether a link is essential or not. The HSS is defined as the collection of links that accumulate nears≈1. Upper and lower insets depict, respectively, the degree distributionp(k) of the HSSs and mean next-neighbour degree kknnl as a function of node degreek. The HSS degree distribution is typically scale-free (seeSupplementary Fig. S2) and the skeletons are typically strongly disassortative. Note that although they may be, and often are, divided into multiple components, the largest connected component of the skeleton typically dominates. This connectedness is not imposed, but is an emergent property of salience. (SeeSupplementary Table S2). We define the salience S of a network as Figure 2: Computation of link salience and properties of the HSS. ( a ) For each reference node r in the weighted network on the left, the SPT T ( r ) is computed. The superposition of all trees according to equation (1) assigns a value s ij to each link in the original network. Salience values are shown on the right with link colour: red is high salience and grey is low. ( b ) The collection of high-salience links (red) for the networks shown in Fig. 1 . The full networks are shown in grey. ( c ) The relative frequency p ( s ) of non-zero salience values s . The distribution p ( s ) is bimodal in all networks under consideration. This key feature of bimodality of p ( s ) provides a plausible, parameter-insensitive classification of links, salient ( s ≈1) versus non-salient ( s ≈0), and implies that nodes in these networks typically agree whether a link is essential or not. The HSS is defined as the collection of links that accumulate near s ≈1. Upper and lower insets depict, respectively, the degree distribution p ( k ) of the HSSs and mean next-neighbour degree k k nn l as a function of node degree k . The HSS degree distribution is typically scale-free (see Supplementary Fig. S2 ) and the skeletons are typically strongly disassortative. Note that although they may be, and often are, divided into multiple components, the largest connected component of the skeleton typically dominates. This connectedness is not imposed, but is an emergent property of salience. (See Supplementary Table S2 ). Full size image so that S is a linear superposition of all SPTs. S can be calculated efficiently using a variant of a standard algorithm (see Supplementary Methods ). According to this definition, the element 0≤ s ij ≤1 of the matrix S quantifies the fraction of SPTs the link ( i , j ) participates in. As T ( r ) reflects the set of most efficient paths to the rest of the network from the perspective of the reference node, s ij is a consensus variable defined by the ensemble of root nodes. If s ij =1, then link ( i , j ) is essential for all reference nodes, if s ij =0 the link has no role and if, say, s ij =1/2 then link ( i , j ) is important for only half the root nodes. Note that although S is defined as an average across the set of SPTs, it is itself not necessarily a tree and is typically different from known structures such as minimal spanning trees (see Supplementary Fig. S1 , Supplementary Table S3 and Supplementary Methods ). Robust classification of links The most important and surprising feature of link salience is depicted in Fig. 2c . For the representative set of networks, we find that the distribution p ( s ) of link salience exhibits a characteristic bimodal shape on the unit interval. The networks' links naturally accumulate at the range boundaries with a vanishing fraction at intermediate values. Salience thus successfully classifies network links into two groups: salient ( s ≈1) or non-salient ( s ≈0), and the large majority of nodes agree on the importance of a given link. As essentially no links fall into the intermediate regime, the resulting classification is insensitive to an imposed threshold, and is an intrinsic and emergent network property characteristic of a variety of strongly heterogeneous networks. This is fundamentally different from common link centrality measures such as weight or betweenness that possess broad distributions (see Fig. 1b ), and which require external and often arbitrary threshold parameters for meaningful classifications. [32] , [33] The salience as defined by equation (1) permits an intuitive definition of a network's skeleton as a structure, which incorporates the collection of links that accumulate at s ≈1. Fig. 2b depicts the skeleton for the networks of Fig. 1a . For all networks considered, only a small fraction of links are part of the HSS (6.76% for the air traffic network, 6.5% for the food web and 2.39% for the world trade network), and the topological properties of these skeletons are remarkably generic. Note that technically a separation of links into groups according to salience requires the definition of a threshold (e.g., we chose the centre of the salience range for convenience). The important feature is that the resulting groups are robust against changes in the value, as almost no links fall into intermediate ranges. Consequently the point of separation is almost arbitrary, yields almost identical skeletons for threshold ranges of 80% of the entire range. One of the common features of these skeletons is their strong disassortativity, irrespective of the assortativity properties of the corresponding original network (see Table 1 ). Furthermore, all skeletons exhibit a scale-free degree distribution Table 1 Statistical features of the full empirical networks and their high-salience skeletons. Full size table with exponents 1.1 ≤ β HSS ≤ 2.5 (see Table 1 and Supplementary Fig. S2 ). As only links with s ≈1 are present in the HSS, the degree of a node in the skeleton can be interpreted as the total salience of the node. The collapse onto a common scale-free topology is particularly striking as the original networks range from quasiplanar topologies with small local connectivity (the commuter network) to completely connected networks (worldwide trade). Note that the lowest exponent (weakest tail) is observed for the commuter network, as in a quasiplanar network the maximum number of salient connections is limited by the comparatively small degree of the original network. The scale-free structure of the HSS consequently suggests that networks that possess very different statistical and topological properties and that have evolved in a variety of contexts seem to self-organize into structures that possess a robust, disassortative backbone, despite their typical link redundancy. Although these properties of link salience are encouraging and suggest novel opportunities for filtering links in complex weighted networks, for understanding hidden core sub-structures and suggest a new mechanism for defining a network's skeleton, a number of questions need to be addressed and clarified for the approach to be viable. First, a possible criticism concerns the definition of salience from SPTs, which suggests that s ij can be trivially obtained from link betweenness b ij , for example, by means of a non-linear transform. Second, a bimodal p ( s ) may be a trivial consequence of broad weight distributions, if for instance large weights are typically those with s ≈1. Finally, the observed bimodal shape of p ( s ) could be a property of any non-trivial network topology such as simple random weighted networks. In the following, we will address each of these concerns. Salience and betweenness The betweenness b ij of a link ( i , j ) is the fraction of all ∼ N 2 shortest paths that pass through the link, whereas the salience s ij is the fraction of N SPTs T ( r ) the link is part of. Despite the apparent similarity between these two definitions, both quantities capture very different qualities of links, as illustrated in Fig. 3 . Betweenness is a centrality measure in the traditional sense [40] , and is affected by the topological position of a link. Networks often exhibit a core-periphery structure [41] and the betweenness measure assigns a greater weight to links that are closer to the barycentre of the network [39] . Salience, on the other hand, is insensitive to a link's position, acting as a uniform filter. This is illustrated schematically in the random planar network of Fig. 3a . High betweenness links tend to be located in the centre of the planar disk, whereas high salience links are distributed uniformly. A given shortest path is more likely to cross the centre of the disk, whereas the links of a SPT are uniformly distributed as they have to span the full network by definition. A detailed mathematical comparison of betweenness and salience is provided in the Methods. Fig. 3c depicts the typical relation of betweenness and salience in a correlogram for the worldwide air traffic network. 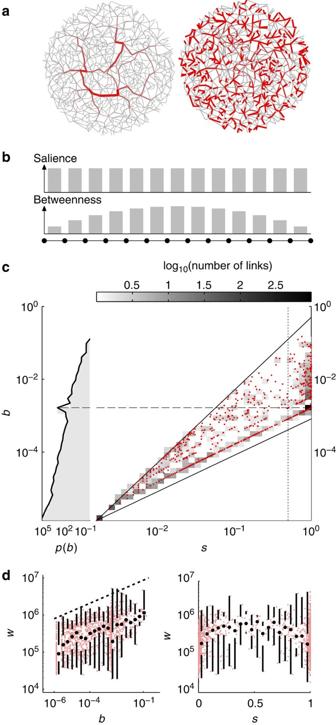Figure 3: Salience and betweenness capture different aspects of centrality. (a) A schematic planar network in which the colour of links quantifies betweennessb(left) and saliences(right). High betweenness links tend to be located near the barycentre of the network,39whereas high-salience links are distributed evenly throughout the network. (b) A simple linear chain shows the reason for this effect. A link in the centre serves as a shortest-path bridge between all pairs of nodes, and so has the highest betweenness. But as all SPTs are identical, all links have identical salience. (c) A scatter plot (red dots) of link saliencesversus link betweennessbfor the air traffic network (point density is quantified in grey). The vertical dotted line markss=1/2 and the solid curves represent the theoretical bounds of equation (3). The projected densityp(b) is shown on the left. The lack of any clear correlation in the scatter plot is typical of all networks inFig. 1(SeeSupplementary Fig. S3for additional correlograms.) (d) Scatter plots (in light red) of betweennessb(left) and saliences(right) versus link weightwin the air traffic network. The bottom and top of the lower whiskers, the dot, and the bottom and top of the upper whiskers correspond to the 0, 25, 50, 75, and 100th percentiles, respectively. The dashed line indicates a scaling relationshipw∼bγwithγ≈0.2. Although the network exhibits a positive correlation between link weight and link betweenness, the HSS incorporates links with weights spanning the entire range of observed values; no clear correlation of weight with salience exists. These properties are observed in the other networks as well. The data cloud is broadly distributed within the range of possible values given by the inequalities (see Supplementary Methods ) Figure 3: Salience and betweenness capture different aspects of centrality. ( a ) A schematic planar network in which the colour of links quantifies betweenness b (left) and salience s (right). High betweenness links tend to be located near the barycentre of the network, [39] whereas high-salience links are distributed evenly throughout the network. ( b ) A simple linear chain shows the reason for this effect. A link in the centre serves as a shortest-path bridge between all pairs of nodes, and so has the highest betweenness. But as all SPTs are identical, all links have identical salience. ( c ) A scatter plot (red dots) of link salience s versus link betweenness b for the air traffic network (point density is quantified in grey). The vertical dotted line marks s =1/2 and the solid curves represent the theoretical bounds of equation (3). The projected density p ( b ) is shown on the left. The lack of any clear correlation in the scatter plot is typical of all networks in Fig. 1 (See Supplementary Fig. S3 for additional correlograms.) ( d ) Scatter plots (in light red) of betweenness b (left) and salience s (right) versus link weight w in the air traffic network. The bottom and top of the lower whiskers, the dot, and the bottom and top of the upper whiskers correspond to the 0, 25, 50, 75, and 100th percentiles, respectively. The dashed line indicates a scaling relationship w ∼ b γ with γ ≈0.2. Although the network exhibits a positive correlation between link weight and link betweenness, the HSS incorporates links with weights spanning the entire range of observed values; no clear correlation of weight with salience exists. These properties are observed in the other networks as well. Full size image Within these bounds no functional relationship between b and s exists. Given a link's betweenness b , one generally cannot predict its salience and vice versa. In particular, high salience links ( s ≈1) possess betweenness values ranging over many scales. The spread of data points within the theoretical bounds is typical for all the networks considered (see Supplementary Fig. S3 ). Links tend to collect at the right-hand edge, corresponding to the upper peak in salience, and in particular at the lower right corner of the wedge-shaped region, corresponding to the heretofore unexplained peak in betweenness exhibited by several of the networks (cf. Fig. 1 and the dashed line in Fig. 3b ). These edges have a maximal salience (all nodes agree on their importance) but the smallest betweenness possible, given this restriction (they are not well represented in the set of shortest paths). Such edges are the spokes in the hub-and-spoke structure: they connect a single node to the rest of the network, but are used by no others, and they are an essential piece of the HSS, as severing them removes some node's best link to the main body of the network. The presence of such links in the HSS explains why the weight values of s ≈1 edges span such a wide range, as a link may have relatively low weight and yet be some node's most important connection. Fig. 3d tests the hypothesis that strong link weights may yield strong values for salience. We observe that link betweenness is positively correlated with link weight and roughly follows a scaling relation w ∼ b γ with γ ≈0.2, in agreement with previous work on node centrality [42] . This is not surprising as high weight links are by definition shorter and tend to attract shortest paths. In contrast, link weights exhibit no systematic dependence on salience, and in particular large weights do not generally imply a large salience. In fact, for fixed link salience the distribution of weights is broad with approximately the same median. Consequently, salience can be considered an independent centrality dimension that measures different features than correlated centrality measures such as weight and betweenness. Origin of bimodal salience All the networks we consider feature broad link weight distributions p ( w ) (see Fig. 1b ), some of which can be reasonably modelled by power laws p ( w ) ∼ w −(1+ α ) with exponents for many empirical data sets typically in the range 1< α <2 (ref. 38 ) (smaller α corresponds to a broader p ( w )). Although it may seem plausible that strong links in the tail of these distributions dominate the structure of SPTs and thus cause the characteristic bimodal distribution of link salience, evidence against this hypothesis is already apparent in Fig. 3d : links with high salience exhibit weights across many scales, and in particular low weight links may possess high salience. Further evidence is provided in Fig. 4a , which depicts the salience distribution for fully connected networks for a sequence of exponent α . For values of α in the range observed in real networks, p ( s ) is peaked near s =0 and decreases with increasing s . A bimodal distribution of s only emerges when α is unrealistically small ( α <1), and is much less pronounced than in real networks (cf. Fig. 2 ). We conclude that broad, scale-free weight distributions p ( w ) alone are insufficient to cause the natural, bimodal distribution p ( s ) observed in real networks. 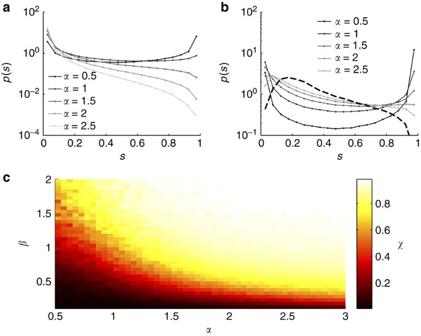Figure 4: Salience in random networks. (a) Salience distributionsp(s) in fully connected networks with 1,000 nodes and weights assigned using a power lawp(w)∼w−(1+α) for various tail exponentsα. Complete networks serve as models of systems with all-to-all interactions, such as the inter-industry trade network. Only for unrealistically broad weight distributions (α≲1), doesp(s) exhibit a bimodal character. Ifα>1, bimodality is absent. (b) Salience distributions in preferential attachment networks (1,000 nodes)23with degree distributionp(k)∼k−3and uniform weights do not exhibit bimodal salience (heavy dashed line). If however the power-law weight distribution is superimposed on the preferential attachment topology, bimodal salience emerges for realistic values ofα. (c) For the range of tail exponentsαandβ, the colour code quantifies the magnitudeχof bimodality in the salience distributionpα,β(s) of a network, with a scale-free degree distribution with exponentβ(constructed using the configuration model4) and a scale-free weight distribution with exponentα. Small values ofχcorrespond to a bimodalpα,β(s). The bimodality measureχwas computed using Kolmogorov–Smirnov distance betweenpα,β(s) fors>0 and the idealized reference distributionq(s)=δ(s−1). Figure 4: Salience in random networks. ( a ) Salience distributions p ( s ) in fully connected networks with 1,000 nodes and weights assigned using a power law p ( w ) ∼ w −(1+α ) for various tail exponents α . Complete networks serve as models of systems with all-to-all interactions, such as the inter-industry trade network. Only for unrealistically broad weight distributions ( α ≲ 1), does p ( s ) exhibit a bimodal character. If α >1, bimodality is absent. ( b ) Salience distributions in preferential attachment networks (1,000 nodes) [23] with degree distribution p ( k ) ∼ k − 3 and uniform weights do not exhibit bimodal salience (heavy dashed line). If however the power-law weight distribution is superimposed on the preferential attachment topology, bimodal salience emerges for realistic values of α . ( c ) For the range of tail exponents α and β , the colour code quantifies the magnitude χ of bimodality in the salience distribution p α,β ( s ) of a network, with a scale-free degree distribution with exponent β (constructed using the configuration model [4] ) and a scale-free weight distribution with exponent α . Small values of χ correspond to a bimodal p α,β ( s ). The bimodality measure χ was computed using Kolmogorov–Smirnov distance between p α,β ( s ) for s >0 and the idealized reference distribution q ( s )= δ(s −1). Full size image Another potential source of the observed bimodality in p ( s ) is the topological heterogeneity of a scale-free degree distribution p ( k ) ∼ k −(1+ β ) with 0< β ≤2 [22] , [23] , [43] . Fig. 4b provides evidence that also a scale-free topology alone does not yield the characteristic bimodal salience distribution. In fact, the generic preferential attachment network [23] ( β =2) with uniform weights exhibits a distribution of salience that is almost the complement of the observed pattern with mostly intermediate values of link salience. The presence of hubs implies that any shortest paths seeking out a node in a hub's region will most likely route through that hub, and links emanating from this hub are more likely to appear in many SPTs. However, the hub-and-spoke structure of a preferential attachment network is only approximate; nodes that are at the end of a spoke are still likely to have random links to other areas of the network. For this reason, it is not typical in the uniform-weight preferential attachment network to find links that appear in nearly all SPTs. However, the observed bimodal distribution p ( s ) can be generated in random networks by a combination of weight and degree variability, a property characteristic of the class of networks discussed here. Fig. 4b also depicts p ( s ) for preferential attachment networks that possess a scale-free distribution of both degree k and weight w . As the weight distribution becomes broader (decreasing α ), and even in the absence of explicit degree–weight correlations, we see the emergence of bimodality in the salience distribution in these networks. Topological hubs are more likely to have extremely high-weight links simply because they have more links. Even when there is a topologically short path terminating at a spoke node that does not pass through the corresponding hub, it is less likely to be the shortest weighted path. Extreme weights amplify the effects of hubs by drawing more shortest paths through them. Moreover, Fig. 4c demonstrates that the emergence of bimodal salience does depend on the interplay between degree and weight distributions: the broader the degree distribution, the narrower the required weight distribution. All of these results support the conclusion that a bimodal salience distribution is the characteristic of networks with strong heterogeneity in both topology and interaction strength, but that unweighted networks do not exhibit this property. Applications to network dynamical systems The relevance of link salience to dynamical processes that evolve on networks is an important issue, and one area of particular interest in network research is contagion phenomena. In this context, individuals in a population are represented by nodes and interaction propensities between pairs of nodes by a weighted network. Contagion phenomena are modelled by transmissions between nodes along the links of the network, where the likelihood of transmission is quantified by the link weights. The central question in this class of models is how the topological properties of the network shape the dynamics of the process. Link salience can also provide useful information about the behaviour of such a dynamical system. To illustrate this, we consider a simple stochastic susceptible-infected (SI) epidemic model. At any given point in time, an infected node i can transmit a disease to susceptible nodes at a rate determined by the link weight w ij . The details of the model are provided in Methods. We consider an epidemic on a planar disk network similar to that shown in Fig. 3a . A single node is chosen at random for the outbreak location. At every step of the process, each infected node randomly selects a neighbour to infect with probability proportional to the link weight; eventually the entire network is infected. By keeping track of which links were used in the infection process, one obtains the infection hierarchy H , a directed tree structure that represents the epidemic pathway through the network. As the process is stochastic, each realization of the process generates a different infection hierarchy. For different initial outbreak nodes and realizations of the process, we calculate an infection frequency h for each link: the number of times that link is used in the infection process, normalized by the number of realizations. The question is how successfully can link salience, a topological quantity, predict infection frequency h , a dynamic quantity. Fig. 5 shows the results for the two different link weight scenarios described in Methods. The top panel shows networks with link weights narrowly and uniformly distributed around a constant value w 0 ; in the bottom panel link, weights are broadly distributed according to a power law. In both cases, link salience is highly correlated with the frequency of a link's appearance in infection hierarchies h , whereas alternative link centrality measures such as weight and betweenness are not (see Fig. 5 insets and Supplementary Information ). The link salience on average gives a much more accurate prediction of the virulence of a link than other available measures of centrality, suggesting that this type of completely deterministic, static analysis could nonetheless have an important role in considering how best to slow spreading processes in real networks. 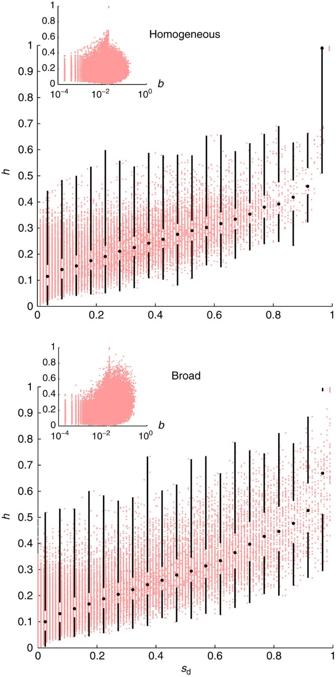Figure 5: Salience predicts infection pathways in stochastic epidemic models. The scatter plots show the directed saliencesdagainst the normalized frequency of appearance in infection pathwayshfor each link in an ensemble of 100 networks, averaged over 1,000 epidemic realizations for each member of the ensemble. As inFig. 3, the plots are divided horizontally into bins, with the heavy black lines indicating quartiles within each bin. Insets show link betweennessbversush, and correlation coefficients are listed inTable 3. Top, Weights distributed narrowly and uniformly around a constantw0. bottom, Weights distributed according top(w)∼w−(1+β)withα=2. Figure 5: Salience predicts infection pathways in stochastic epidemic models. The scatter plots show the directed salience s d against the normalized frequency of appearance in infection pathways h for each link in an ensemble of 100 networks, averaged over 1,000 epidemic realizations for each member of the ensemble. As in Fig. 3 , the plots are divided horizontally into bins, with the heavy black lines indicating quartiles within each bin. Insets show link betweenness b versus h , and correlation coefficients are listed in Table 3 . Top, Weights distributed narrowly and uniformly around a constant w 0 . bottom, Weights distributed according to p ( w ) ∼ w −(1+ β ) with α =2. Full size image As much recent work in network theory has shown [19] , [20] , [31] , [32] , there is tremendous potential for extracting heretofore hidden information from the complex interactions between the elements of a system. However, until now these methods have relied on externally imposed parameters or null models. Here we have shown that typical empirical networks taken from a variety of fields do in fact permit the robust classification of links according to the node-consensus procedure we introduce, and that this leads naturally to the definition of a HSS in these networks. Because vanishingly few links in empirical networks have intermediate values of salience, the identification of the skeleton is insensitive to a salience threshold; indeed, if a tunable filtering procedure is desired other methods may be more appropriate. Not all networks possess a skeleton; simple unweighted models have a shortest-path structure spread throughout the links. However, the presence of a skeleton is a generic feature of many heterogeneously weighted, empirical networks. We suggest that the likely cause in real networks is a hub-and-spoke topological structure along with a broad weight distribution, which amplifies the tendency of hubs to capture shortest paths. We believe that the concept of salience and the HSS will become a vital component in understanding networks of the type discussed here and the development of network-based dynamical models. The simple SI model we investigate here is only a starting point; it may be possible to leverage knowledge of a network's HSS to develop dynamical models that do not require simulation on (or even knowledge of) the full network. The generic bimodal salience distribution in this context also implies that in contagion phenomena, only a small subset of links might typically be active even if the process is stochastic. Those links, however, are almost certainly active irrespective of the outbreak location and the stochasticity of the process, which implies that in this regime the process becomes more predictable and the impact of stochasticity is decreased. This effect may shed a new light on the impact of stochastic factors in disease dynamical processes that evolve in strongly heterogeneous networks. Many of the networks we considered evolved over long periods of time subject to external constraints and unknown optimization principles. The discovery that pronounced weight and degree heterogeneity, which are defining properties of the investigated networks, go hand in hand with generic properties in their underlying skeleton indicate that looking for common evolution principles could be another promising direction of further research. Network data sources Table 2 gives a brief definition of each network we examine here, and below we provide a summary of the networks along with data sources and references. Table 2 Definition of nodes and links in empirical networks. Full size table The Cash flow network was constructed from data collected through the Where's George bill-tracking website ( http://www.wheresgeorge.com ). The nodes are the 3,106 counties in the 48 United States excluding Alaska and Hawaii, and the links measure the number of bills passing between pairs of counties per time. This network has been previously analysed [6] , [10] , [26] ; see in particular the supplement to Thiemann et al . [6] for a wealth of detailed information regarding the construction and statistics of this network, as well as strong evidence for interpreting it as proxy for individual mobility. The network of cash flow is constructed from ∼ 10 million individual bank notes that circulate in the United States. The Air traffic network measures global air traffic based on flight data provided by OAG Worldwide Ltd. ( http://www.oag.com ) and includes all scheduled commercial flights in the world. Nodes represent airports worldwide. Link weights measures the total number of passengers traveling between a pair of networks by direct flights per year. This network is well-represented in the literature [8] , [9] , [25] , [43] , [44] ; we reduce it to 95% flux as described in Woolley-Meza et al . [45] Total traffic in this network amounts to ∼ 3 billion passengers per year. The Shipping network quantifies international marine freight traffic based on data provided by IHS Fairplay ( http://www.ihs.com/products/maritime-information/index.aspx ) which includes itineraries for 16,363 container ships. Nodes represent ports, and links measure the number of commercial cargo vessels traveling between those ports during 2007. The network is available at http://www.mathmod.icbm.de/45365.html and further discussion can be found in Kaluza et al . [46] The Commuting network is based on surveys conducted by the US Census Bureau during the 2000 census, and reflects the daily commuter traffic between US counties; the data is publicly available at http://www.census.gov/population/www/cen2000/commuting/files/2KRESCO_US.zip . Nodes in this network represent the counties of the 48 states excluding Alaska and Hawaii, and links measure the number of people commuting between pairs of counties per day. The Neural network is derived from the Caenorhabditis elegans nematode. Nodes represent neurons, and links measure the number of synapses or gap junctions connecting a pair of neurons. Experimental data is described in White et al . [47] and analysed in Watts and Strogatz [48] ; the network is available at http://www-personal.umich.edu/mejn/netdata/ . The metabolic network measures interactions in the bacterium Escherichia coli [16] , [49] . Nodes represent metabolites and links measure effective kinetic rates of reactions a pair of metabolites participates in. We use only the largest connected component of this network. The Food web network is a representative food web from a list of publicly available data sets of the same type (see http://vlado.fmf.uni-lj.si/pub/networks/data/bio/foodweb/foodweb.htm for networks in Pajek format, a report [50] on trophic analysis of the Florida Bay food web available at http://www.cbl.umces.edu/atlss/FBay701.html and Serrano et al . [32] and Radicchi et al . [33] ). Nodes represent species in the Florida Bay ecosystem, and links measure the consumed biomass in grams of carbon per year across a link. In the Inter-industry network, nodes represent industrial sectors in the United States and their connections are computed from input-output tables prepared by the US Bureau of Economic Analysis available at http://www.bea.gov/industry/io_benchmark.htm . We use data from 2002, the most recent year for which measurements are available. Nodes in this network represent particular industries (for example, 'tobacco production' or 'cutlery and hand tool manufacturing') and links measure an average interaction between two industries. Given two industries x and y , input-output data measures the amount (United States dollars, USD) of input x demands from y to produce one dollar of output, and we take the weight of the link connecting x and y to be the geometric mean of the input-output demand of x on y and y on x . The World trade network is based on data prepared by the United States National Bureau of Economic Research and measures the value (in nominal thousands of USD) of goods traded between countries from 1962 to 2000. Nodes represent countries and links measure the value of goods traded between countries. The data and extensive documentation are available at http://www.cid.econ.ucdavis.edu/data/undata/undata.html . A series of papers analyses a similar data set from a different source [33] , [51] , [52] , [53] . The Collaboration network is based on coauthorship of academic papers in the high-energy physics community from 1995 to 1999. Nodes represent individuals and links measure the number of papers coauthored [54] . The data is publicly available at http://www-personal.umich.edu/mejn/netdata/ . Link salience and betweenness centrality Link salience s and betweenness centrality b are based on the notion of shortest paths in weighted networks. Given a weighted network defined by the weight matrix w ij (not necessarily symmetric) and a shortest path that originates at node x and terminates at node y it is convenient to define the indicator function A shortest path tree T ( x ) rooted at node x can be represented as a matrix with elements and salience s ij of link i→j is given by where 〈·〉 v denotes the average across the set of root nodes x . Betweenness, on the other hand, is defined according to where 〈 · 〉 V 2 denotes the average over all N 2 pairs of terminal nodes. The relation of betweenness and salience can be made more transparent by rewriting this expectation value as a sequential average over all nodes, with fixing root node x . Thus, b ij ( x ) is the conditional betweenness of link i → j if the set of shortest paths is restricted to those terminating at x . From this it follows that Comparing (5) with (4) we see that the difference of salience and betweenness is equivalent to the difference in the shortest path trees T ij ( x ) and the conditional betweenness b ij ( x ), whereas all links in the SPT are weighted equally, links with non-zero conditional betweenness tend to become less central as the links become further separated from the root node x . Formally, we can write with Θ( x )=1 if x >0 and Θ( x )=0 otherwise. Epidemic simulations To determine the relevance of link salience to contagion phenomena on networks, we investigated the correlation of link salience and the frequency at which links participate in a generic contagion process that spreads through planar, random triangular networks. Each network consists of N =100 nodes distributed uniformly at random in a planar disk; the links of the network are given by the Delaunay triangulation of the nodes. The planar distance between nodes is roughly proportional to the number of links in a shortest (network) path between them. A representative example of this type of topology is shown in Fig. 3a . We consider two different weight scenarios: 1 Quasi-homogeneous weights: Each link is assigned a unit weight w modified by an additive, small perturbation ξ where ξ is uniformly distributed in the interval (−0.01, 0.01) 2 Broadly distributed weights: Each link is assigned a random weight from the distribution with PDF We simulate a stochastic SI epidemic process. A single stochastic realization of the process is generated as follows: given a network represented by the symmetric weight matrix w ij , which quantifies the interaction strength of a pair of nodes, we define the probability P ij that node j infects node i in a fixed time interval Δ t where γ ≪ 1/Δ t is the infection rate and Time proceeds in discrete steps; at each step each infected node j chooses an adjacent node to infect at random with probabilities given by P ij . If node j infects a susceptible node i , then the link ( j , i ) is added to the infection hierarchy H , which can be represented as a matrix H ji . In the long-time limit, every node is infected, and H is a tree structure recording the first infection paths from the outbreak location s to every other node. For a given network, we compute R =1,000 different epidemic realizations with random outbreak locations s k , resulting in an ensemble of infection hierarchies H ( k ) mn. The key question is, how frequently does a link in the network participate in an epidemic, and we define the infection frequency of a link as We compute the infection frequency for 100 random networks under each weight scenario, and Fig. 5 illustrates the degree to which the directed salience s mn is a predictor of the dynamic quantity h mn . The correlation of h mn with directed salience and the two measures of centrality we consider here, weight w mn and betweenness b mn , is shown in Table 3 . Table 3 Correlation of other measures with infection frequency. Full size table How to cite this article : Grady, D. et al . Robust classification of salient links in complex networks. Nat. Commun. 3:864 doi: 10.1038/ncomms1847 (2012).